Almost quantum correlations Quantum theory is not only successfully tested in laboratories every day but also constitutes a robust theoretical framework: small variations usually lead to implausible consequences, such as faster-than-light communication. It has even been argued that quantum theory may be special among possible theories. Here we report that, at the level of correlations among different systems, quantum theory is not so special. We define a set of correlations, dubbed ‘almost quantum’, and prove that it strictly contains the set of quantum correlations but satisfies all-but-one of the proposed principles to capture quantum correlations. We present numerical evidence that the remaining principle is satisfied too. Ever since its conception, quantum mechanics has eluded consensual understanding. This has motivated the search for models alternative to quantum theory that could offer a more intuitive explanation of the observed phenomena. The study of modifications of quantum theory has also been motivated by the difficulty in merging it with relativity, the hope being that alternative models may facilitate this task. However, up to now, the existing alterations of quantum theory, even if a priori simple, have been problematic for fundamental reasons. For instance, they have been shown to imply a significant increase in the computational power of the theory [1] or violations of the no-signalling principle [2] , [3] : one of the pillars of relativity that states that superluminal communication is impossible. These results, among others, have led researchers to question whether ‘quantum mechanics is special’ [4] and ‘an island in theory space’ [5] . The possibility that quantum mechanics could indeed be the ultimate physical theory has motivated many attempts to reconstruct it from physically intuitive axioms within the framework of generalized probabilistic theories [6] , [7] , [8] , [9] . All such works, however, rely on a separation between states and observables, implicit in the formalism of generalized probabilistic theories. Furthermore, most axioms in this research programme are formulated in terms of abstract entities, such as states, which are not directly testable in an experiment. A different approach was introduced in ref. 10 , where the authors propose to classify and study physical theories according to the correlations that they allow to generate between different systems. In this approach, the goal is to understand quantum correlations from physical principles stated only in terms of correlations. The advantage of this approach comes from the fact that correlations among systems can be experimentally estimated in a ‘device-independent’ way, that is, just from the observed statistics and without any theoretical modelling of the systems. Thus, contrary to the axioms in the reconstruction paradigm, the validity of device-independent principles can be put to test without further considerations. Popescu and Rohrlich [10] initiated this research line by considering whether quantum theory is the most nonlocal theory compatible with special relativity. They initially conjectured that, if Nature were more nonlocal, then we could violate special relativity just as observed in the aforementioned modifications to quantum theory. Remarkably, they proved that the answer to this question is negative and one can posit the existence of non-quantum but also non-signalling correlations [10] . Even though the principle of no-signalling fails to capture quantum correlations, the work of Popescu and Rohrlich motivated the quest to find a principle that does. As a result, several device-independent principles have been proposed so far that have been partly successful at capturing the nonlocality of quantum physics [10] , [11] , [12] , [13] , [14] , [15] . As above, the hope is to prove that the presence of correlations beyond quantum theory would have implausible consequences, in the sense of violating a reasonable principle for physical correlations, providing an intuitive explanation for the degree of nonlocality in quantum theory. It is worth mentioning that the programme of understanding quantum correlations is vast and has been considered from different perspectives. For instance, in contextuality scenarios, quantum correlations refer to those correlations observed among different projective (or sharp) measurements subject to some compatibility constraints (see, for instance, refs 16 , 17 , 18 for different formalizations of contextuality scenarios). Here, we follow Popescu and Rohrlich and focus on correlations among outputs of measurements performed on separate systems. Note also that we do not consider sequences of measurements; therefore, measurements produce one single classical output. It is then assumed that no communication takes place among the systems while the measurements are performed, which can be enforced by arranging the measurements so that they define space-like separated events. As mentioned, and contrary to other approaches, the virtue of the considered scenario is that correlations can be estimated in a device-independent manner. In this work, we show that quantum theory is, at the level of correlations among systems, not as special as expected. In particular, we identify a set of non-signalling correlations, which we name ‘almost quantum’, and prove that this set (i) is strictly larger than the set of quantum correlations but (ii) satisfies all-but-one of the device-independent principles proposed for quantum correlations. Moreover, we offer strong evidence that it satisfies the remaining principle too. Our results demonstrate that it is possible to modify the structure of quantum correlations without running into any operational contradiction with quantum predictions. They also shed doubts on the research programme of recovering quantum correlations from ‘natural’ device-independent physical principles. Finally, invoking arguments from the history approach introduced in the context of quantum gravity, we motivate the study of almost quantum correlations as a possible avenue for generalizations of quantum theory. The set of almost quantum correlations The considered scenario consists of n different parties each having access to a system, or box in what follows, see Fig. 1 . Each j th party, for j ε{1, 2,..., n }, inputs a classical symbol x j from a set of M possible inputs into his box and as a result receives one output a j ε{0, 1,..., d −1}. Thus, every scenario is labelled by these possible values as an ( n , M , d ) scenario. The correlations observed in this scenario are described by the ( dM ) n conditional probabilities of observing outputs when using inputs . They can be collected into a vector of ( dM ) n positive numbers, which satisfy normalization over all d n outputs (for each of the M n choices of inputs). Since it is assumed that the different processes are local, that is, that the systems do not exchange any communication when producing the outputs given the inputs, the observed correlations must satisfy the no-signalling principle. 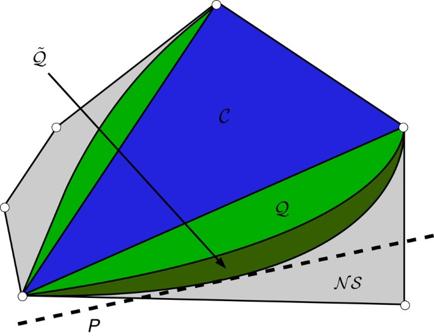Figure 1: Sets of correlations in a device-independent setting. In this work we study the sets of correlations produced by space-like separated boxes (inset) each with an inputajand outputxj. All sets of correlations outside of the space of classical correlations labelledare nonlocal correlations and all correlations within the set labelledsatisfy special relativity. The set of quantum correlations is then. We introduce a set that is an extension to quantum mechanics: the set of ‘almost quantum’ correlations. This principle implies that for all permutations (and relabelling of the parties after permutation) of n parties Figure 1: Sets of correlations in a device-independent setting. In this work we study the sets of correlations produced by space-like separated boxes (inset) each with an input a j and output x j . All sets of correlations outside of the space of classical correlations labelled are nonlocal correlations and all correlations within the set labelled satisfy special relativity. The set of quantum correlations is then . We introduce a set that is an extension to quantum mechanics: the set of ‘almost quantum’ correlations . Full size image where the left-hand-side is a sum over m ≤ n parties. In other words, the marginal conditional probability distributions are well defined for all possible subsets of parties. The linear constraints (1) define the set of non-signalling correlations, denoted by , see Fig. 1 . The no-signalling constraints can, for instance, be enforced by arranging the input–output processes so that they define space-like separated events. The set of quantum correlations, denoted by , represents a strict subset of non-signalling correlations [10] , [19] . They are defined as those conditional probability distributions that can be generated by the Born rule as where: (1) | ψ › is a normalized vector in a finite dimensional Hilbert space ; (2) are projectors acting on and defining the measurements by each party, that is, and , the identity matrix; (3) any two measurement operators of two different parties commute, . Note that in this work quantum correlations are defined using the commuting measurement paradigm rather than the tensor product of local measurements. This is because in the commuting measurement paradigm the comparison with almost quantum correlations (defined in what follows) becomes more transparent. Note that the two paradigms are known to be equivalent for finite dimensional systems, while the equivalence for infinite dimensions remains open [20] . Hence, by demanding to be finite dimensional, all our results remain unchanged when switching to the tensor product representation. After these preliminaries, we are now in position to define the set of almost quantum correlations, denoted by . This set is defined by those correlations which can be written as where (1) | ψ › is a normalized vector in a Hilbert space ; (2) are projectors acting on and defining the measurements by each party, that is, and , the identity matrix; (3) one has for any arbitrary permutation π of the n parties. We provide an alternative definition of the set of almost quantum correlations in terms of efficiently solvable semi-definite programmes (see Methods and Supplementary Note 1 ). For two parties the set of almost quantum correlations coincides with the set of correlations satisfying the 1+AB level of the Navascués–Pironio–Acin (NPA) hierarchy for quantum correlations [20] , known as Q 1+AB . Correlations in Q 1+AB have already been shown as useful as quantum correlations for certain information-processing tasks [21] , [22] . When defining a set of non-signalling correlations, the first natural requirement to be met is that the set remains stable under post-processing. That is, it should be impossible to generate correlations outside the set by combining correlations within the set. The natural set of operations when dealing with correlated systems, or boxes, is given by post-selection, wirings of the boxes and distribution of boxes among parties (and the combinations of all of them), see Fig. 2 . While this consistency requirement may seem trivial at first sight, and in fact it holds for classical, quantum and non-signalling correlations, it is not satisfied in general [23] . We prove that the set of almost quantum correlations is stable under classical post-processing (see Supplementary Note 2 ). 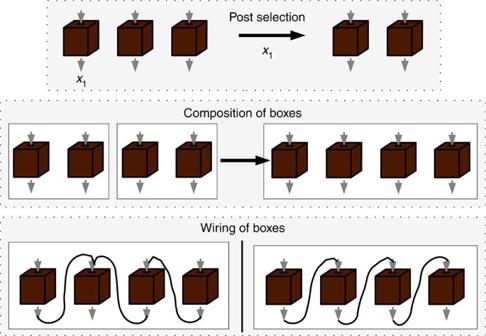Figure 2: Closure under classical post-processing operations. In order for a set of non-signalling correlations to be consistent, they need to be stable under classical post-processing. That is, given some boxes that produce correlations in a given set we should not be able to leave this set after classical post processing (resulting in new correlations) on the measurement data. All classical post-processing can be reduced to: (1) post selection (looking at correlations conditioned on a particular output of another box); (2) grouping of two sets of boxes to make a new set of boxes; and (3) wiring the boxes together so that inputs to some boxes are dependent on the outputs of others. We can also perform logical operations on the classical data to choose which form of post processing to perform. We show that if correlations belong to the almost quantum setthen any classical post processing on these correlations will result in new correlations that are also inside(Supplementary Note 2). Therefore, the almost quantum set is stable under classical post processing. Figure 2: Closure under classical post-processing operations. In order for a set of non-signalling correlations to be consistent, they need to be stable under classical post-processing. That is, given some boxes that produce correlations in a given set we should not be able to leave this set after classical post processing (resulting in new correlations) on the measurement data. All classical post-processing can be reduced to: (1) post selection (looking at correlations conditioned on a particular output of another box); (2) grouping of two sets of boxes to make a new set of boxes; and (3) wiring the boxes together so that inputs to some boxes are dependent on the outputs of others. We can also perform logical operations on the classical data to choose which form of post processing to perform. We show that if correlations belong to the almost quantum set then any classical post processing on these correlations will result in new correlations that are also inside ( Supplementary Note 2 ). Therefore, the almost quantum set is stable under classical post processing. Full size image Quantum versus almost quantum correlations It is already clear from the definitions that the set of quantum correlations is included in the set of almost quantum correlations. In fact, this inclusion can be proven to be strict; thus, . First of all, there already exist numerical results proving the existence of bipartite supraquantum correlations , which satisfy the step 1+AB of the NPA hierarchy, see for instance refs 20 , 24 . In what follows, we provide an analytical proof of this strict inclusion already in the simplest possible case of two observers performing two measurements of two outputs. Consider a Bell scenario as in Fig. 1 with two inputs a k ε{0, 1}, two outputs x k ε{0, 1} and two parties ( k =1, 2). Owing to normalization and no-signalling constraints, any probability distribution in this scenario can be written as an eight-dimensional vector where p i ( α | β ) is the probability p ( a i | x i ) where a i = α and x i = β . In this scenario, one can define the following Bell-like expression built from a linear combination of the observed probabilities , with The minimum of this quantity over quantum correlations is slightly larger than −1 (see Supplementary Note 3 ), that is, is an inequality satisfied by quantum correlations. This inequality can be violated by almost quantum correlations. We can provide an example of almost quantum correlations such that (see Supplementary Note 3 ). This value is smaller than the quantum minimum, and thus . The discrepancy between quantum and almost quantum correlations is in principle experimentally testable. For instance, the previous Bell-type inequality for quantum correlations can be tested as the standard Clauser–Horne–Shimony–Holt Bell inequality [25] in an experiment involving two measurements of two outputs on two different systems. More in general, any Bell inequality whose maximal quantum violation is not obtained at the 1+AB level of the NPA hierarchy provide experimental tests between quantum and almost quantum correlations. As mentioned, examples of these inequalities can be found in refs 20 , 24 . Of course, what is not possible at the moment is to think of a concrete experimental set-up in which this test could in principle be performed. Note that just defines a set of correlations, and not a complete physical theory, with well-defined state space, dynamics and measurements, which one can use to describe physical set-ups and whose correlation structure coincides with the set of almost quantum correlations. Thus, although from we can assert that, for some nonlocality experiments, the almost quantum set predicts violations of the quantum bounds, the lack of a physical theory prevents us from proposing an explicit experiment in which this discrepancy could be observed. Device-independent principles Comparing the definitions of quantum and almost quantum correlations, it is clear that the only difference between the two sets appears in the third condition. In the case of almost quantum correlations, rather than demanding full commutation of the measurement operators by the different parties, one imposes the weaker condition that these measurements must commute when acting on the measured state | ψ ›. The intuition behind this definition is that in order to appreciate an operational difference between the two sets, one should probe the non-commutativity of the measurement operators in when acting on states different from | ψ ›. However, it is not clear how to get this information when one has only access to the correlations . On the basis of this intuition, one may expect that the two sets are equivalent for many operational tasks. Our next results show that this intuition is correct: despite the set of almost quantum correlations is strictly larger than the quantum one, almost quantum correlations can be proven to satisfy almost all the device-independent information principles that aim at singlling out the set of quantum correlations. This implies that none of these principles suffice to characterize quantum correlations. To our knowledge, there have been five of such principles: Non-trivial Communication Complexity (NCC) [11] , No Advantage for Nonlocal Computation [12] , Information Causality (IC) [13] , Macroscopic Locality (ML) [14] and Local Orthogonality (LO) [15] . The first three principles are defined in communication scenarios where two parties, call them Alice and Bob, must evaluate a bivariate function under limited communication or no communication at all. For NCC, Alice and Bob receive, respectively, the n -bit strings . Their task is to compute the binary function with just one bit of communication. In this context, NCC postulates that there does not exist a universal number such that any function can be computed with worst-case probability greater than p , see Fig. 3 . For NANLC, the scenario is as follows: a referee randomly generates two bit strings , according to the probability distributions (uniform) and , respectively. The referee then sends Alice (Bob) the string , and Alice and Bob’s task is to produce a pair of bits a , b such that . Alice and Bob are thus carrying out a particular type of distributed computation. Their performance is limited by the principle of NANLC, which states that, no matter what type of nonlocality resources Alice and Bob share, their average success probability for computing function f should not beat the classical value. IC requires Alice (Bob) to be distributed a random n -bit string (a random number k ε{1, ..., n }). Here both parties must cooperate so that Bob ouputs a bit b with b = x k , and Alice is allowed to send Bob m bits of communication. 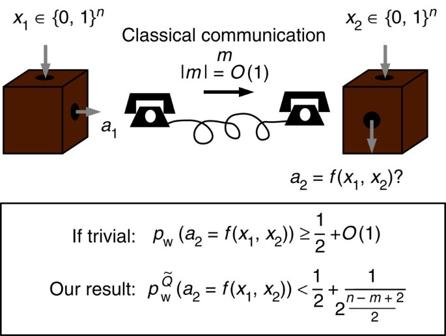Figure 3: The communication complexity scenario. The possibility of correlations more nonlocal than quantum, allowing for trivial communication complexity, was first highlighted in ref.39. This observation was turned into the principle of NCC11and applies to the scenario of probabilistic communication complexity tasks. In this scenario, two parties, labelled 1 and 2, are each given a (generally different) input bit stringx1andx2, respectively, of lengthnand after receiving these inputs party 1 receives an outputa1from their resources and communicates some number of bits to party 2 and party 2 outputsa2. We assume that the number of bits is a constant |m|=O(1). The most general statement we can make of the NCC principle says that no set of correlations will give a worst-case probability of success (for all possible inputs and all possible functions) bounded away from a half by a constant. An important result in our work is that for all correlations in the set, this worst-case probability of success is not bounded away from a half by a constant. The principle of IC claims that the efficiency of the above scheme is subject to the constraint Figure 3: The communication complexity scenario. The possibility of correlations more nonlocal than quantum, allowing for trivial communication complexity, was first highlighted in ref. 39 . This observation was turned into the principle of NCC [11] and applies to the scenario of probabilistic communication complexity tasks. In this scenario, two parties, labelled 1 and 2, are each given a (generally different) input bit string x 1 and x 2 , respectively, of length n and after receiving these inputs party 1 receives an output a 1 from their resources and communicates some number of bits to party 2 and party 2 outputs a 2 . We assume that the number of bits is a constant | m |= O (1). The most general statement we can make of the NCC principle says that no set of correlations will give a worst-case probability of success (for all possible inputs and all possible functions) bounded away from a half by a constant. An important result in our work is that for all correlations in the set , this worst-case probability of success is not bounded away from a half by a constant. Full size image where I (A:B) denotes the mutual information between the random variables A and B [26] . The last two principles, ML and LO, have a somewhat different flavour. For ML, an experimental set-up where two parties carry out extensive measurements over a macroscopic number of independent particle pairs is considered. ML postulates that, under low-resolution detectors (of precision, ), the statistics of such macroscopic experiments should admit a classical—local—description. LO is an intrinsically multipartite physical principle that states that, for any set E of pairwise locally orthogonal, ∑ e ε E p ( e )≤1. Two measurement events are called ‘locally orthogonal’ if k ε{1, ..., n } such that . Before this work, it was known that correlations satisy ML if and only if they satisfy the first step of the NPA hierarchy [14] , the corresponding set being denoted by Q 1 (see Supplementary Note 4 ). Since Q 1+AB is included in Q 1 , almost quantum correlations satisfy ML. The proofs that almost quantum correlations have non-trivial communication complexity provide no advantage for nonlocal computation and satisfy local orthogonality are much more involved (see Supplementary Notes 5 – 7 ). At the moment, we are unable to prove that all almost quantum correlations satisfy IC. We believe that the difficulty in the proof comes from the fact that the entropic-like figure of merit (6) is hard to be bound without appealing to notions more sophisticated than correlation limits alone, such as the von Neumann entropy. However, up to now a series of works has explored the power of IC in different correlation scenarios [13] , [27] , [28] , [29] . We tested almost quantum correlations against all the known bounds and in all the cases we could reproduce or improve them ( Supplementary Note 8 ). Put together, these numerical results strongly suggest that almost quantum correlations satisfy IC too. Most of the existing results on IC have been derived in the case of two parties, as IC was originally defined in this scenario. However, it is possible to extend IC to scenarios involving more than two parties by simply imposing that correlations among N parties satisfy IC whenever they satisfy inequality (6) for any splitting of the parties into two groups. This generalization is analogous to what is done for the no-signalling principle. Adopting this generalization of IC, and using the methods described in ref. 30 , we can show ( Supplementary Note 9 ) that certain three-party almost quantum correlations beyond the quantum theory satisfy IC too (and thus all currently proposed principles). This second result implies that, even when taken together, all these principles are unable to capture quantum correlations, at least in the multipartite setting. This, however, does not exclude the possibility that IC is enough to single out bipartite quantum nonlocality. Almost quantum correlations and the history approach All our previous results have shown that the set of almost quantum correlations is, in terms of the known device-independent principles, as plausible as the quantum set. Thus, so far, we do not have any good reason justifying why correlations inside should not be realizable in Nature. Now, what about correlations outside ? Could we enlarge further without violating basic physical laws? Or, in other words, is there a way of singling out the set of almost quantum correlations? Our last goal is to discuss how it is possible to identify the set of almost quantum correlation using arguments arising from the history approach to quantum gravity. In ref. 31 , Sorkin proves that the dynamics of any history-based physical theory with no third-order interference effects is described by a so-called ‘decoherence functional’, a concept that originated in the decoherent history approach to quantum mechanics (see, for example, refs 32 , 33 , 34 ). The decoherence functional is a matrix whose rows and columns are labelled by histories, and determines which partitions of the set of all possible histories are physically meaningful, together with the probability that the actual history of the universe falls into one of those subsets. In ref. 35 , this general decoherence functional approach is applied to describe bipartite Bell experiments. Interestingly, the authors conclude that, demanding the decoherence functional to satisfy the extra condition of strong positivity (SP), which just means that the decoherence functional is demanded to be a semidefinite positive matrix, the set of accessible two-party correlations precisely corresponds to the 1+AB level of the NPA hierarchy. As shown here, in the case of two parties, this level coincides with the set of almost quantum correlations. While this connection is intriguing, the authors of ref. 35 do not give a strong justification for the SP condition used in its derivation. However, recently, the SP condition has been shown to emerge naturally from the requirement that any history-based theory, possibly supraquantum, should be able to describe single-site quantum experiments. The above results not only imply that almost quantum correlations are compatible with Sorkin’s lack of third-order interference [31] , see also ref. 36 , but also that this principle, together with the need to accommodate single-site quantum experiments in our theory, precludes the existence of correlations outside the set of almost quantum correlations . In this study we have identified a set of correlations, named almost quantum, that, despite being strictly larger than the quantum set, seems to satisfy all device-independent principles proposed so far to single out quantum correlations. This set is consistent and has an efficient numerical characterization. Our results hence suggest that it is possible to modify the correlation structure of the quantum theory without running into any operationally relevant consequence. They also pose a convincing barrier to the research programme that aims to characterize quantum nonlocality, utilizing fundamental principles motivated by physical and information theory perspectives. The set of almost quantum correlations is thus a powerful tool for understanding nonlocality. In view of all these points, it would be interesting to derive a physical theory underpinning . On the one hand, this theory could provide the first reasonable extension of quantum mechanics. As mentioned, so far, any such extension has often led to violations of the no-signalling principle or significant increases of the information power of the theory. A theory explaining almost quantum correlations would not suffer from these problems. On the other hand, this theory could be used to propose concrete experimental set-ups to test those Bell-like inequalities for which quantum and almost quantum correlations predict different bounds. In this regard, it would be tempting to interpret the state and projection operators appearing in the definition of , not as some auxiliary mathematical entities, but as the physical state and measurements of an underlying theory generating the correlations. However, this is just a possibility as valid as any other. In fact, it is unclear to us how to define a reasonable dynamics in this context. Another, possibly more promising, alternative is to search for a theory within the history approach. All these possibilities deserve further investigation but are beyond the scope of the present work. We would like to conclude with an interesting speculation. An important conceptual difference between quantum and almost quantum correlations appears when considering the computational complexity of their characterization. Given some correlations p (a|x), determining whether they are quantum, , or almost quantum, , defines two decision problems. As indicated, the almost quantum problem can be efficiently solved using semidefinite programming techniques. On the contrary, the quantum problem appears to be much harder, as it has been shown that approximating the quantum violation of bipartite Bell inequalities is NP-hard [38] . Actually, it is not even known if the quantum problem is decidable. This raises a very provoking final thought: assume the quantum problem was undecidable, does one expect correlations in Nature to be undecidable? Semidefinite programming and almost quantum correlations In this section we re-express the definition of the set of almost quantum correlations as a semidefinite programme. Let us first introduce some useful terminologies. Given m ≤ n parties, the pair , with the components of labelled by each of the m parties will be called an ‘event’. For example, for n =3, the event ( a 1 , a 3 | x 1 , x 3 ) represents the physical situation in which parties 1 and 3 have measured x 1 , x 3 , and obtained, respectively, the outcomes a 1 , a 3 . Following ref. 15 , we say that two events are ‘locally orthogonal’ (represented ee ′) if there is a common party k such that , and . We now present another useful characterization of the set of all almost quantum distributions. Lemma 1 . if, for any event with for all parties k involved, there exists a vector with the properties (1) , if . (2) , where | φ › is the vector corresponding to the null event, that is, none of the party measures. Note that 1= P ( φ )=‹ φ | φ ›, that is, | φ › is normalized. (3) , where is any event that doesnot involve the measuring parties in the events and . Note that any set of complex vectors subject to restrictions (1), (2), (3) implies the existence of real vectors subject to the same constraints. It follows that, in the above semidefinite programme, all free variables can be taken to be real. Proof . The right implication follows by defining . Regarding the left implication, consider the subspaces . From condition (1), we have that , for a ≠ a ′. It follows that the projectors on the subspaces , that is, satisfy . Now, the action of on the vector | φ › is given by: where we have used that in order to conclude . The second term vanishes, since by virtue of relation (3). Note that, also by condition (3), the last equality holds when we replace | φ ›, | a k , x k › by , , where is any event where party k does not intervene. It follows that . By induction, we thus arrive at for , where the product is taken in whatever order. Finally, define From equation (8) and relation (2) it thus follows that the state | φ › and the operators satisfy the conditions required to produce almost quantum correlations. Given this lemma, we are now in a position to give the semidefinite programming version of almost quantum correlations. By the Gram decomposition [38] , the existence of a set of vectors satisfying the conditions of Lemma 1 is equivalent to the existence of a positive semidefinite matrix Γ, with rows and columns labelled by events with for all parties involved, and such that · , where is any event not involving the measuring parties in the events and . We call any such matrix Γ an ‘almost quantum certificate’ for . How to cite this article: Navascués, M. et al . Almost quantum correlations. Nat. Commun. 6:6288 doi: 10.1038/ncomms7288 (2015).